Pseudomonas aeruginosaadaptation in the nasopharyngeal reservoir leads to migration and persistence in the lungs Chronic bacterial infections are a key feature of a variety of lung conditions. The opportunistic bacterium, Pseudomonas aeruginosa , is extremely skilled at both colonizing and persisting in the airways of patients with lung damage. It has been suggested that the upper airways (including the paranasal sinuses and nasopharynx) play an important role as a silent reservoir of bacteria. Over time, P. aeruginosa can adapt to its niche, leading to increased resistance in the face of the immune system and intense therapy regimes. Here we describe a mouse inhalation model of P. aeruginosa chronic infection that can be studied for at least 28 days. We present evidence for adaptation in vivo , in terms of genotype and phenotype including antibiotic resistance. Our data suggest that there is persistence in the upper respiratory tract and that this is key in the establishment of lung infection. This model provides a unique platform for studying evolutionary dynamics and therapeutics. Chronic airway infections are common in a variety of patient groups including those with bronchiectasis [1] , late stages of chronic obstructive pulmonary disease [2] and cystic fibrosis (CF) [3] . CF is an autosomal recessive disorder affecting 1 in 25,000 people in the United Kingdom and 1 in 30,000 in the United States. The genetic disorder leads to abnormal ion transport across cell membranes making CF a multiorgan disease. In the lungs, this leads to impaired mucociliary clearance, altered cilia beating and chronic lung infection. Chronic lung infection in CF patients is a debilitating condition, giving rise to progressive and extensive lung damage eventually leading to patient death. P. aeruginosa is the major cause of chronic lung infection and by adulthood up to 80% of patients are infected [4] . Although early-eradication therapy has shown some success in clearing initial P. aeruginosa infection, patients often develop chronic infections that are impossible to eradicate. Several studies have investigated changes in diversity and adaptation of P. aeruginosa during long-term lung infections [5] , [6] , [7] ; however, there is a relative lack of knowledge concerning the initial stages of infection. This can be explained, in part, by the difficulty in obtaining such samples from patients. A study by Li et al . [8] showed that 29% of CF patients acquired P. aeruginosa in the first 6 months of life. Despite these obstacles, there would be clear health and economic benefits to intervention at this important step in CF respiratory microbiology [9] . During chronic infection, P. aeruginosa grows as a biofilm and displays both extensive diversification and antimicrobial resistance [6] , [7] . However, the exact route from environmental microorganism to lung pathogen is unclear. The upper respiratory tract, including the nasopharynx and paranasal sinuses, has been identified as a potential reservoir for P. aeruginosa. Sinus complications, including chronic sinusitis, have been reported in CF patients [10] . Furthermore, P. aeruginosa has been identified in these sinusitis samples [11] and similarities between the isolates found in the paranasal sinuses and the lungs have been observed [10] , [12] . In a study by Muhlebach et al . [13] , P. aeruginosa isolates were recovered more frequently from the sinuses than from bronchoalveolar lavage fluid of CF patients. It has been suggested that colonization of the upper reaches of the respiratory tract (including the nasopharynx and paranasal sinuses) allows P. aeruginosa to adapt to the anoxic environment present in the lower lung [14] . Following this, adapted bacteria can descend along the respiratory tract and cause lung infection and chronic inflammation. While many groups have described murine models of P. aeruginosa respiratory infection, these are often acute pneumonia models that result in either rapid bacterial clearance or development of sepsis and host death [15] . Longer-term models also exist, which use agar beads impregnated with bacteria to mimic chronic infection [15] . However, these models do not allow the study of the early stages of infection nor do they closely reflect the natural respiratory route of infection. Transmissible strains of P. aeruginosa have been reported worldwide [16] . The Liverpool Epidemic Strain (LES) is a widespread transmissible strain that has been associated with increased patient morbidity and mortality [17] . We have reported previously that different subtypes of the same strain can exhibit highly different infection characteristics [18] . Here we exploit these characteristics to develop a novel murine respiratory inhalation model whereby P. aeruginosa is introduced intranasally and establishes stable colonization of the nasopharynx and infection of the lungs over a 28-day period. Early gene expression and adaptation are studied and compared with behaviour in an established in vitro model of P. aeruginosa biofilm formation. We show that bacteria introduced via a natural inoculation establish colonization in the nasopharynx enabling adaptation and migration down into the lungs. In addition, we demonstrate that P. aeruginosa -adapted isolates display a significant increase in their ability to colonize the murine respiratory tract. P. aeruginosa abundance in the murine respiratory tract To assess the levels of P. aeruginosa LESB65 in the murine lung during initial colonization, mice were inoculated intranasally and tissue samples were analysed at various time points to determine both the bacterial numbers and variations in gene expression. Numbers of P. aeruginosa were highest in both the lung and upper respiratory tract (referred to hereafter as nasopharynx, but that also includes the paranasal sinuses) immediately after infection (a mean colony forming unit (CFU) per mg tissue of 1,604 for the nasopharynx and 6,007 for the lung; all bacterial counts were derived from five mice per time point). Over the first 12 h, there was a period of decrease in the bacterial numbers present in both infection sites (to 397 CFU per mg nasopharynx, 190 CFU per mg lung). Post 12 h, P. aeruginosa levels in the nasopharynx and lungs began to increase, with higher numbers present in the nasopharynx up to 72 h post infection (782–970 CFU per mg nasopharynx between 24 and 72 h). Post 72 h, a significant decrease in P. aeruginosa CFU in the nasopharynx (<0.05) and lungs ( P <0.001) was observed (177 CFU per mg nasopharynx and 1 CFU per mg lung at 168 h; Fig. 1a ). 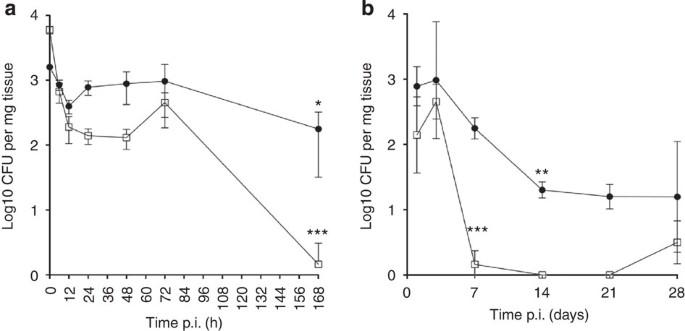Figure 1:P. aeruginosain the murine lung and nasopharynx. P. aeruginosacolony forming units present in the lung (white squares) and nasopharynx (black circles) of mice following intranasal inoculation with LESB65 over (a) 7 days (168 h) and (b) 28 days. Data shown are the mean and s.d. of five or more mice per group per time point. Significant differences are denoted by an asterisk determined using a two-way ANOVA and relate to differences as compared with the previous time point. *P<0.05, **P<0.01, ***P<0.001. Figure 1: P. aeruginosa in the murine lung and nasopharynx. P. aeruginosa colony forming units present in the lung (white squares) and nasopharynx (black circles) of mice following intranasal inoculation with LESB65 over ( a ) 7 days (168 h) and ( b ) 28 days. Data shown are the mean and s.d. of five or more mice per group per time point. Significant differences are denoted by an asterisk determined using a two-way ANOVA and relate to differences as compared with the previous time point. * P <0.05, ** P <0.01, *** P <0.001. Full size image The murine infection model was extended over a longer time period to determine whether P. aeruginosa could be maintained in the respiratory tract beyond 7 days ( Fig. 1b ). P. aeruginosa persisted in the nasopharynx for the 28-day period of the experiment, with a gradual decrease in CFU observed between 7 and 14 days post infection (from 776 CFU per mg nasopharynx on day 7 to 20 CFU per mg on day 14), with bacterial numbers stabilizing thereafter (19 CFU per mg on day 21 and 16 CFU per mg on day 28). P. aeruginosa was undetectable in the lungs by day 14. Interestingly, however, on day 28, P. aeruginosa was isolated from the lungs of all of mice tested (mean 26 CFU per lung). Diagnostic PCR tests were used to confirm that the isolates were the LES, suggesting that long-term persistence in the nasopharynx allowed reseeding of the lower respiratory compartment ( Fig. 1b ). Early changes in gene expression In order to study changes in gene expression during the early stages of infection, genes involved in biofilm formation and virulence were targeted. During the initial 7-day experiment, the gene expression of P. aeruginosa detected in the lung varied over time ( Table 1 ). At 6 h, genes associated with early biofilm formation flgD , algD and pelB showed increases (more than twofold) in expression, with algD displaying more than sixfold increase in expression. Expression levels of these genes then decreased over time. Expression of pelB only was greater than twofold increased at 72 h. Gene expression data for 168 h in the lung were not available because the numbers of P. aeruginosa were too low. In the nasopharynx, algD, flgD, lasR and pelB were all upregulated during the 168-h period. The quorum sensing-associated gene, lasR , showed the highest upregulation, with a >30-fold increase in expression 168 h after inoculation. Although there was limited similarity in the gene expression profiles of the lung and nasopharynx, perhaps reflecting the different metabolic requirements of the two compartments, both samples showed upregulation of algD 6 h post infection and upregulation of pelB at 72 h post infection. The gene expression profiles were also compared with expression detected in an in vitro artificial sputum biofilm model over the same time period ( Table 1 ). In this model, unlike the murine model, expression of rhlR and phzF was detected. Some similarities across the different sample types were detected. pelB expression was common to all three sample types and the nasopharynx and artificial sputum medium (ASM) samples showed similar levels of flgD expression at 168 h post infection ( Table 1 ). Table 1 Ranking of the 21 key TFs identified by master regulator analysis. Full size table Adaptation in the respiratory tract Five P. aeruginosa isolated from the nasopharynx of each mouse on days 1, 3, 7, 14, 21 and 28 were subjected to further study to determine whether phenotypic changes could be detected. In addition, isolates from the lungs on day 28 were studied to determine whether differences between isolates from the nasopharynx and lungs could be detected at the end of the experiment. Using growth during the log phase to calculate the fitness of each population, it was evident that the fitness decreased over time, with isolates from populations sampled on days 3, 7, 14, 21 and 28 showing significantly decreased fitness compared with the original LESB65 isolate ( Fig. 2 ). 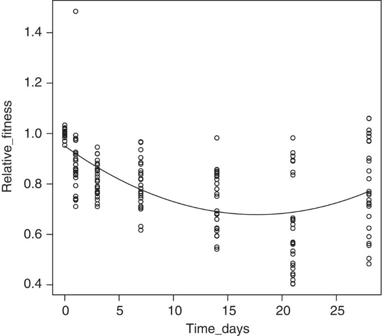Figure 2: Changes in the fitness in Luria broth (LB) ofP. aeruginosapopulations from the nasopharynx of mice over time points up to 28 days post-inoculation. At each time point, measurements from 25 isolates (derived from five mice) were determined in triplicate. Statistical analysis was performed in R using a linear mixed effect model to determine the effect of time on fitness. Time was a significant factor (P≤0.001). Figure 2: Changes in the fitness in Luria broth (LB) of P. aeruginosa populations from the nasopharynx of mice over time points up to 28 days post-inoculation. At each time point, measurements from 25 isolates (derived from five mice) were determined in triplicate. Statistical analysis was performed in R using a linear mixed effect model to determine the effect of time on fitness. Time was a significant factor ( P ≤0.001). Full size image Antibiotic susceptibility tests using the disk diffusion method were performed on all isolates. Increased resistance to tobramycin was evident as a step-wise development of smaller zones of inhibition, and a significant difference was detected by days 21 and 28 ( Fig. 3a ). In addition to the significant difference, the mean zone size of inhibition on days 21 and 28 was below 19 mm, the cutoff for tobramycin resistance used in diagnostic laboratories [19] . Therefore, during the 28-day infection period, the bacteria changed from tobramycin-sensitive to -resistant in the absence of antibiotic pressure. For ciprofloxacin, significantly smaller zone sizes were detected on days 1, 3, 7, 14 and 21 compared with the day-0 isolates. However, there was no significant difference on day 28 ( Fig. 3b ). 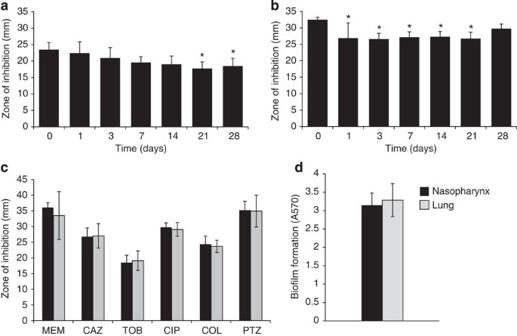Figure 3: Changes in antimicrobial susceptibility ofP. aeruginosaisolates isolated from the nasopharynx. (a) Resistance to tobramycin in isolates from the nasopharynx over 28 days. (b) Resistance to ciprofloxacin in isolates from the nasopharynx over 28 days. (c) Comparison of antibiotic resistance of isolates derived from the nasopharynx (black) and lung (grey) on day 28. (d) Comparison of surface-attached biofilm formation of isolates derived from the nasopharynx (black) and lung (grey) on day 28. At each time point, measurements from 25 isolates (derived from five mice) were obtained in triplicate for the disk diffusion tests and from eight replicates for the biofilm formation assay. The mean and s.d. are shown. Significant differences were determined using Kruskal–Wallis one-way analysis of variance on Ranks and Dunn’s method. Statistically significant differences from time zero are denoted with *P≤0.01. MEM-meropenem, CAZ-ceftazidime, TOB-tobramycin, CIP-ciprofloxacin, COL-colistin, PTZ-piperacillin/tazobactam. No significant differences in susceptibility to any of the six antibiotics tested were detected between isolates derived from the nasopharynx and lungs on day 28 ( Fig 3c,d ). Figure 3: Changes in antimicrobial susceptibility of P. aeruginosa isolates isolated from the nasopharynx. ( a ) Resistance to tobramycin in isolates from the nasopharynx over 28 days. ( b ) Resistance to ciprofloxacin in isolates from the nasopharynx over 28 days. ( c ) Comparison of antibiotic resistance of isolates derived from the nasopharynx (black) and lung (grey) on day 28. ( d ) Comparison of surface-attached biofilm formation of isolates derived from the nasopharynx (black) and lung (grey) on day 28. At each time point, measurements from 25 isolates (derived from five mice) were obtained in triplicate for the disk diffusion tests and from eight replicates for the biofilm formation assay. The mean and s.d. are shown. Significant differences were determined using Kruskal–Wallis one-way analysis of variance on Ranks and Dunn’s method. Statistically significant differences from time zero are denoted with * P ≤0.01. MEM-meropenem, CAZ-ceftazidime, TOB-tobramycin, CIP-ciprofloxacin, COL-colistin, PTZ-piperacillin/tazobactam. Full size image The genome sequences of 10 isolates from the nasopharynx and 10 isolates from the lung on day 28 were compared with the original LESB65 isolate used to infect the mice at the start of the model. Ninety-four single-nucleotide polymorphisms (SNPs) were detected between LESB65 and the reference genome LESB58 ( Supplementary Data 1 ). All of these SNPs were also identified in a previous sequencing study [20] . Only one additional SNP was detected in multiple isolates, a non-synonymous SNP resulting in a missense mutation in pmrB ( Supplementary Data 1 and Fig. 4 ). Isolates with this mutation were found both in the nasopharynx and the lungs. Further screening using PCR amplicon sequencing ( Table 2 ) revealed that this mutation was present in 3/25 isolates isolated from the nasopharynx on day 21 from three separate mice. Two isolates derived from the same mouse, with and without the pmrB mutation (NP22_2 and NP22_4, respectively), were selected for rechallenge infection experiments in the mouse model to assess whether adaptation influenced the capacity of LESB65 to establish chronic infection. 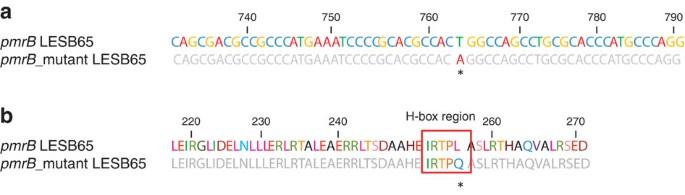Figure 4: Single-nucleotide polymorphism in the sequence of thepmrBgene ofP. aeruginosa. (a) DNA sequence of a portion of thepmrBgene showing wild-type LESB65 and the mutation found in three isolates using genome sequencing. (b) Translated amino-acid sequence of the same region ofpmrBfrom wild-type and mutant LESB65. Changes from the wild-type sequence are denoted with *. Figure 4: Single-nucleotide polymorphism in the sequence of the pmrB gene of P. aeruginosa . ( a ) DNA sequence of a portion of the pmrB gene showing wild-type LESB65 and the mutation found in three isolates using genome sequencing. ( b ) Translated amino-acid sequence of the same region of pmrB from wild-type and mutant LESB65. Changes from the wild-type sequence are denoted with *. Full size image Table 2 Primers used in this study. Full size table Rechallenge experiment using evolved isolates Three isolates were used in the mouse model over a 7-day period to determine differences in their ability to persist; LESB65 (original isolate), NP22_2 ( pmrB mutation present) and NP22_4 (no pmrB mutation), the latter two were isolated from the same mouse on day 21. These two isolates did not differ significantly from each other in all other traits measured including growth, biofilm formation, antibiotic resistance and colony morphology. Colony counts from the nasopharynx and lung were performed on mice rechallenged with these strains. In the nasopharynx, NP22_2 had significantly higher CFU on day 1 (mean 1,259 CFU per mg) and 7 (870 CFU per mg) compared with the original LESB65 (575 CFU per mg and 174 CFU per mg on days 1 and 7, respectively), while NP22_4 had significantly higher CFU on days 1 (1,778 CFU per mg), 2 (1,786 CFU per mg), 3 (1,428 CFU per mg) and 7 (1,223 CFU per mg) post rechallenge. Overall, CFU levels for both isolates (NP22_2 and NP22_4) were significantly higher than the original LESB65 isolate by day 7 ( Fig. 5a ). In the lungs, the NP22_2 isolate clearly outperformed the original LESB65 isolate at every time point and by day 7 it was detected at levels approximately three logs higher than the original isolate (mean 5,464 CFU per mg for NP22_2 versus 3 CFU per mg for LESB65; Fig. 5b ). The NP22_4 isolate showed significantly higher levels on days 1 (89125 CFU per mg versus 243 CFU per mg) and 2 (28183 CFU per mg versus 195 CFU per mg) (compared with the original isolate); however, there was no significant difference from day 3 onwards. Thus, evolved isolates clearly outperformed the original LESB65 isolate in vivo . 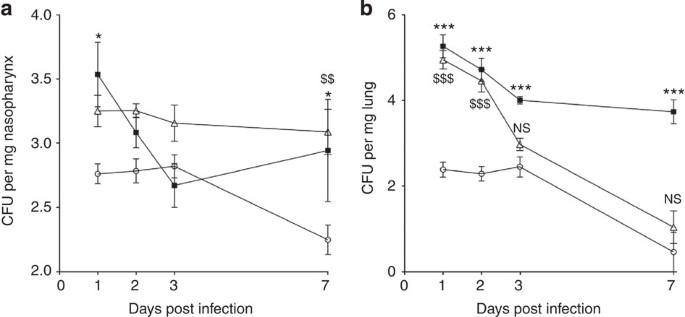Figure 5:P. aeruginosaadapted isolates in the murine lung and nasopharynx. Rechallenge experiment using isolates derived from day 21 of the mouse infection model in (a) the nasopharynx and (b) the lungs. Isolates from the same mouse with thepmrBmutation (NP22_2, black squares) and without it (NP22_4, white triangles) were compared with the original LESB65 input isolate (white circles). * and $ refer to statistically significant differences in two-way ANOVA with Bonferroni post test for LESB65 versus NP22_2 (*) and NP22_4 ($).*P<0.05,
    P<0.01,***/
$P<0.001, NS=not significant. Figure 5: P. aeruginosa adapted isolates in the murine lung and nasopharynx. Rechallenge experiment using isolates derived from day 21 of the mouse infection model in ( a ) the nasopharynx and ( b ) the lungs. Isolates from the same mouse with the pmrB mutation (NP22_2, black squares) and without it (NP22_4, white triangles) were compared with the original LESB65 input isolate (white circles). * and $ refer to statistically significant differences in two-way ANOVA with Bonferroni post test for LESB65 versus NP22_2 (*) and NP22_4 ($). * P <0.05, 
    P <0.01, ***/
$ P <0.001, NS=not significant. Full size image In this study, we describe a novel murine model of P. aeruginosa infection that can be studied over at least 28 days. The bacteria are introduced via a natural inoculation (inhalation) route leading to stable colonization of the nasopharynx. This allows seeding down into the lungs over an extended period of time and P. aeruginosa was detected in all the mice on day 28. To our knowledge, this is the first model of P. aeruginosa infection to describe such persistence, adaptation and migration. Both phenotypic and genotypic changes in isolates recovered from mice were detected, showing that P. aeruginosa adapts rapidly to its in vivo environment. When adapted isolates were used to rechallenge the respiratory system, both adapted isolates displayed a significant increase in their ability to colonize the nasopharynx when compared with the ancestral isolate. Furthermore, the isolate (NP22_2) carrying a genetic mutation in a regulator gene, pmrB , also showed a significant increase in its ability to persist in the lungs after 7 days. Adaptive changes in this isolate led to a four-log increase in CFUs in the lungs on day 7. These results not only highlight an exciting, new model in which potential novel therapeutics could be tested over a longer infection period, but also provide important data on the early, adaptive changes that P. aeruginosa can undergo. This reinforces the notion that the upper respiratory tract, including the nasopharynx, plays a vital role in the establishment and persistence of infection. Murine models have been used previously to study both acute and chronic infection with P. aeruginosa . Acute pneumonia models often use intranasal or intratracheal inoculation resulting in either rapid clearance or acute sepsis and death [15] . Chronic infection models, using both mice and rats, have traditionally used immobilizing methods such as impregnating the bacteria into agar beads resulting in longer-term infection and similar properties to the human clinical situation [15] , [21] . However, it has been demonstrated that the spread of bacteria to the alveoli is difficult to achieve when beads are used [22] and that alginate beads may cause mechanical blocking and damage to the bronchi [23] . Whereas models utilizing intranasal infection have often been associated with acute pneumonia [15] , a mouse model resulting in a 7-day infection has been reported previously [22] . Here we show that intranasal infection can also be applied to the establishment of longer colonization/infection, representing a chronic situation. Differences in susceptibility to bacteria have been reported between different mouse strains [15] and we have also shown previously that different isolates of the same strain can respond differently in these animal models [18] . Hence, both the mouse and bacterial strain used are clearly important factors in the establishment of clinically relevant infection models. In this study, the combination leads to a model that uses both a natural route of inoculation (inhalation) and a longer time period of infection and therefore offers an ideal platform for studying the establishment of long-term respiratory tract infections. This study shows that, in this model, P. aeruginosa can stably colonize the murine upper respiratory tract, including the nasopharynx and paranasal sinuses, for at least 28 days. In addition, the route of administration used represents a natural route of infection via nasal inhalation as opposed to the use of agar beads. We demonstrate clearly that P. aeruginosa is extremely adept at colonizing the nasopharyngeal niche. The link between the microbiology of the upper and lower respiratory tracts has been the subject of a number of studies [11] , [13] , [24] , [25] . A study by Johansen et al . [26] showed that in intermittently colonized CF patients, 91% were found to carry identical P. aeruginosa genotypes in the sinuses and lungs, suggesting that the sinuses could be a reservoir for both adaptation and repeated infection/colonization of the lungs. Furthermore, the same study showed that adaptation in the upper reaches of the respiratory tract would differ to that in the lungs because of an altered immune response. Whereas the immune response in the lung is characterized by polymorphonuclear leucocytes and inflammation, the response in the sinuses is characterized by IgA, which has anti-inflammatory properties [14] , [26] , [27] . Studies have shown that CF patients with persistent P. aeruginosa in the sinuses often have a distinct lack of systemic antibody responses, thus questioning the current definition of chronic infection [12] , [26] , [27] . In addition to the altered immune response in these different niches, ciliary beat frequency has also been found to be altered in nasal airway cultures leading to significantly more P. aeruginosa attaching to these cultures than tracheal airway cultures [28] , therefore showing that mucociliary clearance is not uniform throughout the respiratory tract and may contribute to persistence in the upper reaches of the airways. Ciliary function is further impaired in CF patients and this may contribute to the unique susceptibility of CF patients to chronic P. aeruginosa infections. In our murine model, we have demonstrated that there are no significant differences in phenotype in isolates from the nasopharynx and lungs after 28 days in the lung. Furthermore, we detected changes in the genotype in isolates from both the nasopharynx and the lungs showing that the presence of the pmrB mutation was not restricted to a single niche. This is consistent with the hypothesis that isolates from the nasopharynx seed into the lungs to aid in the establishment of infection. Previously, it has been difficult to assess the directionality of movement of bacteria between the upper and lower respiratory tracts; however, the high levels of P. aeruginosa in the nasopharynx in this model support the idea of downwards migration suggested by others [12] , [26] , [29] The importance of nasopharyngeal colonization is highlighted by other respiratory pathogens such as Streptococcus pneumoniae [30] . The exact mechanism of migration remains unclear. Both aspiration due to viral infection or during sleep have been suggested [12] , [31] , with the latter seemingly more likely in this study. Sinonasal persistence has also become an important consideration in patients undergoing lung transplantation. It has been reported that donor lungs can become colonized within 4 weeks with P. aeruginosa that has an identical genotype to pretransplant lung isolates [32] . The upper respiratory tract including the nasopharynx and paranasal sinuses are clearly important as potential reservoirs. Our novel model addresses this relatively understudied but key niche. A further feature of chronic P. aeruginosa infections, particularly those associated with CF patients, is adaptation over time [5] . Adaptation in populations of P. aeruginosa from patients has previously been demonstrated in terms of colony morphology, growth, antibiotic resistance, mucoidy, biofilm ability and motility [5] , [33] . The biofilm mode of growth is a key feature in persistent, chronic lung infections and facilitates the development of adaptation and diversity [34] . The bacteria grow in multicellular communities surrounded by an exopolysaccharide matrix and P. aeruginosa growing as a biofilm expresses certain genes, including algD, pel and psl [34] , [35] . We investigated a small subset of these genes involved in biofilm formation and virulence to determine whether expression was upregulated in this model. Alginate is an important exopolysaccharide produced by P. aeruginosa and most commonly associated with the mucoid phenotype. High levels of algD expression were detected in both respiratory niches 6 h after infection and, in the nasopharyngeal samples, the fold change in gene expression remained high over the first 72 h. LESB65 is a nonmucoid isolate that has recently been genome-sequenced [20] . It has been shown previously that nonmucoid isolates display increased levels of algD expression in both a mouse model and in the lungs of CF patients [36] . Growth under anaerobic conditions was found to be a key trigger in alginate gene expression [36] , and reduced oxygen availability has been reported in both the CF lung [37] and the upper respiratory tract [14] . Previous studies have reported that the growth conditions present in the agar beads often used in animal models of P. aeruginosa lung infection can induce alginate expression in nonmucoid strains [36] . However, in our model of natural inhalation infection, alginate expression in a nonmucoid strain was observed without the presence of agar beads, and therefore this may be a common feature of respiratory infection. As in previous studies, our findings suggest that alginate is a key virulence factor in the establishment of infection [38] , particularly in the nasopharynx [26] . In addition to alginate, P. aeruginosa also produces other extracellular polysaccharides that can act as a major component of the biofilm matrix, including Pel and Psl. Nonmucoid isolates can use either Pel or Psl as a major polysaccharide providing both a structural scaffold and a protective barrier [39] . Structural redundancy between Pel and Psl has been reported, with different strains relying on different polysaccharides [40] . LESB65 displays upregulation of pel but not psl , a similar expression profile to that seen in PA14 but not PAO1 (ref. 40 ). This upregulation was identified in both the upper and lower respiratory tracts of P. aeruginosa -infected mice as well as an in vitro model using artificial sputum. In chronically infected patients, biofilms have been detected in both the upper and lower respiratory tracts, with the major difference being the level of polymorphonuclear leucocytes around the biofilm (higher levels in the lungs) [26] . The expression of these biofilm-related genes supports previous work where P. aeruginosa has been found to form biofilms in the paranasal sinuses [26] . Biofilm-related genes were expressed in samples from both the upper and lower respiratory tracts of the mice adding to the evidence that P. aeruginosa biofilms form in both niches, again supporting the relevance of this model to the actual clinical state in chronic infections. Upregulation of other genes, including those associated with quorum sensing, was also detected, particularly in the nasopharynx. This suggests high expression of virulence factors in P. aeruginosa nasopharyngeal populations that may aid the bacteria’s ability to persist long term in this niche. We observed adaptive changes in growth fitness and antibiotic resistance over the 28-day period. The growth characteristics of the isolates changed over time, with the initial isolate showing greater fitness for growth in LB during the log phase than isolates from subsequent time points. Lowered fitness of P. aeruginosa isolates growing in laboratory media from CF chronic lung infection has been reported previously [41] . However, here we demonstrate that, over time, the isolates became more adapted to the respiratory tract, as evidenced by the success of later isolates in the rechallenge experiments. These results combined suggest that isolates within these populations became more adapted to the in vivo environment but less successful in the in vitro environment. In this study, changes in antibiotic resistance to tobramycin and ciprofloxacin were observed with isolates becoming significantly more resistant over time. It has been shown that genes associated with multidrug efflux pumps are often upregulated in isolates derived from the paranasal sinuses, and resistance to both of these antibiotics was detected [12] . This altered gene expression in isolates from the upper reaches of the respiratory tract, which then seed down into the lungs, may contribute to the early development of antibiotic resistance. Hoffman et al . [42] found that resistance to these two antibiotics was a common feature of lasR mutants and that these traits can develop in the absence of the antibiotics, primarily driven by metabolic shifts in response to nutrient availability within host tissues. Genome sequencing however did not reveal the presence of mutations in lasR in this study; therefore, the mechanisms underlying these phenotypic changes remain unclear. It has been suggested that the upper respiratory tract, including the nasopharynx and paranasal sinuses, could be an ‘evolutionary nest’ and a ‘silent reservoir’ allowing adaptation to the respiratory tract [26] , [29] . The rechallenge experiments support this by showing that isolates that had evolved in the mouse respiratory tract for 21 days were more successful than the original isolate in re-establishing infection in both upper and lower respiratory tract niches. The apparent increased fitness in the relevant environment suggests the accumulation of beneficial mutations. Using whole-genome sequencing and PCR screening, only one SNP was identified in multiple isolates, in pmrB , resulting in a missense mutation. Studies on the evolution of CF-associated lineages of P. aeruginosa have reported similar mutation rates, estimated at 2.1–2.6 SNPs per year [43] , [44] . Interestingly, a missense SNP in pmrB has also been identified as a fixed, adaptive mutation in the evolutionary history of the CF-associated DK2 lineage of P. aeruginosa [5] . PmrB is a two-component regulator system signal sensor kinase and the mutation identified in this study is contained in the conserved H-box region [45] suggesting that it is likely to have a functional impact. This results in a change from leucine, a non-polar (hydrophobic) amino acid to glutamine, a polar (hydrophilic) amino acid. PmrAB mutants have been linked to resistance to polymyxins and cationic antimicrobial peptides derived from host neutrophils and epithelia [46] . In previous studies, mutations have led to hyperactivation of the pmrAB system and elevated expression of genes involved in lipopolysaccharide modification [47] . The importance of the PmrAB response and associated gene expression has been linked to antimicrobial resistance, including aminoglycoside resistance, in P. aeruginosa biofilms [48] . The isolate carrying this mutation was significantly more successful at colonizing the lungs than another isolate (without the pmrB mutation) isolated from the same mouse at the same time. Both adapted isolates showed higher levels of colonization than the original isolate, suggesting that, although the pmrB mutation may contribute to this effect (particularly in the lungs), other unidentified genetic and epigenetic factors may also play an important role. The natural mutations generated in this model could provide important targets for genotypes that appear to be beneficial in these early stages of infection and establishment in a long-term niche. This study strongly supports the hypothesis that bacterial populations in the upper reaches of the respiratory tract adapt, and that this host niche offers a relatively protected environment for bacterial colonization and adaptation. This model is the first animal model that allows the simultaneous study of both niches through long-term persistence and migration from the upper to the lower respiratory tract. The process of adaptive radiation whereby a variety of phenotypes and genotypes are descended from a single clone [33] , [49] can be modelled and therefore this study provides an exciting and novel platform in which both evolutionary dynamics and efficacy of therapeutics could be studied. Bacterial strains Bacteria were stored at −80 °C in 10% (v/v) glycerol until use. LESB65 was used throughout the study. This isolate has previously been shown to colonize the nasopharynx [18] and has been genome-sequenced [20] . LES isolates were identified by PCR amplifying the two LES markers PS21 and LESF9 (ref. 50 ). Bacteria were routinely grown on Columbia agar or overnight in LB broth at 37 °C and 200 r.p.m. Infection of mice Female BALB/cOlaHsd mice were purchased from Harlan Laboratories (Bicester, UK) and were acclimatized for 1 week before use. Mice used for infection experiments were between 9 and 14 weeks of age and were age-matched for each experiment. The UK Home Office and University of Liverpool ethics committee approved the experimental protocols. Animals were anaesthetized with a mixture of O 2 and isofluorane and infected intranasally with a fresh mid-log phase dose of 2 × 10 6 CFU P. aeruginosa strain LESB65 in 50 μl phosphate-buffered saline (PBS). Mice did not develop visible signs of disease and were culled at pre-determined times post infection (0, 6, 12 h and days 1, 2, 3, 5, 7, 14, 21 and 28). Mice were culled by cervical dislocation, and the lungs and nasopharynx were removed and snap-frozen on dry ice for subsequent RNA extraction or else used for assessment of bacterial colonization and in vivo growth. Gene expression studies and bacterial counts were performed on five mice per time point studied. Mouse group size was calculated using methodology described by Shah [51] for the calculation of sample sizes for dichotomous variables. Bacterial counts Serial dilutions of 20 μl samples (of lung or nasopharynx homogenized in 5 ml PBS) were performed in sterile 96-well microtitre plates (GIBCO, Paisley, UK). Serial dilutions to 10 −7 were made with each sample. Pseudomonas-selective plates (Oxoid, UK) were used to analyse three 20 μl aliquots of each dilution. This procedure was repeated in duplicate. Plates were incubated at 37 °C overnight. Colonies were counted in sectors containing a measurable number (approximately <200). Statistical analysis was performed using a two-way analysis of variance (ANOVA) with Bonferroni post hoc tests in SigmaPlot version 12.0. Population adaptation On days 1, 3, 7, 14, 21 and 28, where possible, five isolates from each of the five mice were isolated and studied to determine changes in phenotypic characteristics. Growth was studied by inoculating one colony into 200 μl of LB medium. Optical density (A600) was measured every 30 min over a period of 46 h using a Fluostar Omega microplate reader (BMG Labtech). Data were analysed using the MARS Data Analysis Software (BMG Labtech). Fitness was calculated as described previously using data from the log phase of growth in the first 12 h [52] . Statistical analysis was performed using a linear mixed effect model to test the effect of time in the nlme package in R. Determination of bacterial colony morphology variants was performed by randomly selecting individual isolates. Isolates were streaked on Columbia agar and incubated for 1–2 days at 37 °C. Biofilm formation of individual isolates was performed as described previously [18] . Briefly, a total of 200 μl of P. aeruginosa culture diluted 1:100 overnight in LB was added to each well. For each isolate, 12 replications were performed. Incubation was carried out at 37 °C for 48 h, after which time the spent culture was removed and the wells were washed three times with PBS. The biofilms were air-dried and quantified using crystal violet staining (at absorbance 570 nm). Results were analysed using Kruskal–Wallis analysis of variance and Dunn’s post hoc test for nonparametric data. Antimicrobial sensitivity testing was performed using the disk susceptibility testing method according to the guidelines of the British Society of Antimicrobial Chemotherapy [19] . The diameter of inhibition zones was recorded and antimicrobial susceptibility was determined according to the zone diameter breakpoints of the British Society of Antimicrobial Chemotherapy. Biofilm formation ability was studied using crystal violet staining as described previously [18] . Statistical analysis was performed using nonparametric ANOVAs and Dunn’s post hoc tests in SigmaPlot version 12.0. P. aeruginosa biofilm formation in artificial sputum medium ASM was prepared as previously described [53] . Briefly, 4 g DNA was added slowly to 250 ml of sterile water; 5 g mucin was dissolved in a further 250 ml of sterile water. Most amino acids (0.25 g each) were dissolved in 100 ml of water. Cysteine was dissolved in 25 ml water and tyrosine in 25 ml of 0.5 M KOH. In all, 5.9 g diethylenetriaminepentaacetic acid, 5 g NaCl and 2.2 g KCl were dissolved in a further 100 ml of water. The DNA, mucin, egg yolk emulsion (5 ml) and amino-acid/salt solutions were combined and adjusted to pH 6.9 with Tris-HCl and made up to a total volume of 1 l with sterile water. This ASM solution was then filter-sterilized. Overnight cultures of bacterial strains were diluted in ASM to an optical density (OD) measured at 600-nm wavelength (OD600) of 0.05 (±0.01). Fresh ASM was inoculated 1:100 with diluted overnight cultures and 2.0 ml cultures/well were grown in 24-well microtitre plates (Iwaki, tissue-culture-treated) for 7 days at 37 °C and 75 r.p.m. Plates were secured with laboratory film (Parafilm) during incubation. Bacteria were analysed at times 0, 6, 12 h, and 1, 2, 3 and 7 days. At each time point, bacterial counts were performed on Columbia agar using serial dilutions and RNA was extracted for analysis of changes in gene expression. For disruption of bacterial biofilms, ASM cultures were mixed with equal volumes of sputasol and incubated for 15–30 min in at 37 °C and 250 r.p.m. shaking. RNA extraction and cDNA synthesis For RNA extraction from ASM, RNAlater (Life Technologies) was added and mixtures were incubated for 5–10 min at room temperature. Bacteria were harvested using centrifugation for 30 min at 2,750 g and 4 °C. Supernatant was removed and bacterial pellets were used for subsequent RNA isolation or stored at −70 °C. For biofilm disruption, 16 ml of Sputasol (Oxoid; prepared in RNase-free water) were added to RNA later -treated ASM cultures and mixtures were incubated for 25–30 min at 37 °C and 250 r.p.m. shaking before centrifugation. RNA from bacterial cultures was isolated using the RNeasy Midi Kit (Qiagen) according to the Protocol for isolation of Total RNA from bacteria (Qiagen). Isolation was performed in an RNase-free environment using RNase-free consumables and RNase-free reagents. Lysozyme (1 mg ml −1 , prepared in RNase-free TE) treatment of bacterial pellets was carried out for 5–7 min at room temperature. Purified RNA was eluted with RNase-free water. For RNA extraction from mouse lungs and nasopharynx, tissue was weighed and immediately homogenized using a high-speed tissue homogenizer. Following this, samples were extracted using the RNeasy Mini Kit (Qiagen). Following RNA extraction, the samples were subjected to treatment with a MicrobEnrich kit (Ambion, Life Technologies) to deplete the eukaryotic RNA from the samples. For all samples, isolated RNA was subsequently DNase-treated using Turbo DNase (Ambion) in order to remove remaining genomic DNA. RNA preparations were analysed for remaining genomic DNA by conventional PCR designed to amplify the reference gene rpoD ( Table 2 ). Quantification of RNA was performed by measuring the absorbance at 260 nm wavelength using the NanoDrop8000 UV–vis Spectrophotometer (Thermo Scientific) and purity of RNA was analysed by determination of the 260/280 nm ratio. Molecular grade water was used as blank. The 260/280 nm ratio obtained for all samples was between 1.7 and 2.1. First-strand cDNA synthesis was performed using the SuperScript II Reverse Transcriptase (Invitrogen) according to the manufacturer’s instructions in an RNase-free environment using RNase-free consumables and RNase-free reagents. Two independent rounds of cDNA synthesis were performed and samples were pooled before further analysis. cDNA was stored at −20 °C until used. Quantitative real-time PCR and gene expression analysis Quantitative real-time PCR (qPCR) was performed using the Rotor-Gene Q cycler (Qiagen) and 0.1-ml strip-tubes (Qiagen). Each 20 μl reaction consisted of 1 × Rotor-Gene SYBR Green PCR Master Mix (Qiagen), specific forward and reverse primers ( Table 2 ), and 2 μl cDNA and molecular grade water added to a final volume of 20 μl. Thermal cycling was carried out as follows: activation of DNA polymerase at 95 °C for 5 min, followed by 40 cycles of 95 °C for 10 s, 60 °C for 15 s and 72 °C for 20 s. Fluorescence data were collected at the end of every 72 °C step. PCR products were subsequently analysed by melting curve analysis ranging from 72 to 95 °C. Each qPCR was performed in triplicate and a standard curve of known copy number was performed in each run. No-template controls were included in each qPCR reaction and contained molecular grade water instead of template DNA. When necessary, qPCR products were analysed using agarose gel electrophoresis. Obtained data were analysed using the Rotor-Gene Q series software (Qiagen). Relative expression levels of genes algD, flgD, lasR , rhlR , phzF , pelB and pslD were calculated using the two-standard curve method. Genes proC and rpoD , encoding the pyrroline-5-carbocylate reductase and sigma factor RpoD, respectively, were used as reference genes. These genes are frequently used for gene expression studies in P. aeruginosa and have been shown to be stable expressed [54] , [55] . Primers used for gene expression analysis are shown in Table 2 . A standard curve was constructed for each target and reference genes. Genome sequencing Isolates were grown overnight in LB media. DNA was extracted using the Wizard Genomic DNA Purification Kit (Promega) and quantified using the Qubit HS assay and a Qubit Fluorometer (Life Technologies). Genomic libraries were prepared using the Nextera XT preparation kit as per the manufacturer’s instructions (Illumina, San Diego). Libraries were sequenced as barcoded pools on the Illumina MiSeq using V2 reagents generating paired sequencing reads of 250 bases in length. Reads were quality-filtered and trimmed for Nextera adaptor sequences using Trimmomatic. Reads were aligned to the P. aeruginosa LESB58 reference sequence (NCBI accession code: NC_011770) using BWA MEM [56] . Alignments were filtered for a minimum mapping quality of 30 and variants were called using VarScan 2.3.5 (ref. 57 ). Variants were filtered by employing a minimum allele frequency of 90%, a P value cutoff of less than 0.05 and with the strand filter enabled, meaning that variants must be supported with evidence from reads in both orientations. The strand filter will ignore variants that have >90% of support from one strand only. Additional data were obtained from the Pseudocap database [58] . Short reads for all samples were deposited in the European Nucleotide Archive (ERP005854). How to cite this article: Fothergill, J.L. et al . Pseudomonas aeruginosa adaptation in the nasopharyngeal reservoir leads to migration and persistence in the lungs. Nat. Commun. 5:4780 doi: 10.1038/ncomms5780 (2014). Accession codes: Short reads for the genomic sequences are deposited in the European Nucleotide Archive with accession code ERP005854 .